Single-shot tomographic movies of evolving light-velocity objects Tomography—cross-sectional imaging based on measuring radiation transmitted through an object along different directions—enables non-invasive imaging of hidden stationary objects, such as internal bodily organs, from their sequentially measured projections. Here we adapt tomographic methods to visualize—in one laser shot—the instantaneous structure and evolution of a laser-induced object propagating through a transparent Kerr medium. We reconstruct ‘movies’ of a laser pulse’s diffraction, self-focusing and filamentation from phase ‘streaks’ imprinted onto probe pulses that cross the main pulse’s path simultaneously at different angles. Multiple probes are generated and detected compactly and simply, making the system robust, easy to align and adaptable to many problems. Our technique could potentially visualize, for example, plasma wakefield accelerators, optical rogue waves or fast ignitor pulses, light-velocity objects, whose detailed space–time dynamics are known only through intensive computer simulations. In the 1870s, English photographer Eadweard Muybridge used an array of cameras activated by trip lines strung across a horse’s path to show that it became temporarily airborne while galloping, thus settling a hotly debated question of his time [1] . Muybridge’s demonstration did not rely on repeatability of the horse’s motion. Rather, he established his point by capturing a series of stop-action frames within one cycle of the horse’s gallop, a few of which revealed the horse’s legs collected beneath its airborne body. In modern science, researchers still seek a method to record a Muybridge-like multiframe movie of evolving light-velocity objects created by laser or charged particle pulses during a single transit through matter. These objects include optical rogue waves used to model giant ocean waves [2] , nonlinear plasma wakes used to accelerate charged particles [3] , fast ignitor pulses used to trigger laser fusion [4] , filamenting laser pulses used for atmospheric analysis [5] and filamenting electron bunches used to model astrophysical jets [6] . Sophisticated single-shot techniques exist for measuring the complete electric field profile E ( z (loc) , x ( ⊥ ) ) (or charge-density profile ρ ( z (loc) , x ( ⊥ ) )) of an ultrashort light [7] , [8] , [9] (electron [10] ) pulse that initiates such events, analogous to the opening frame of Muybridge’s movie. Here, z (loc) = z − vt is the local longitudinal position relative to the centre of the pulse propagating at velocity v , x ( ⊥ ) a vector transverse to the propagation ( z ) axis, z distance into the medium and t time after the pulse enters the medium. However, when the pulse propagates nonlinearly through matter, its profile E ( z (loc) , x ( ⊥ ) , t ) (or ρ ( z (loc) , x ( ⊥ ) , t ))—and the co-propagating refractive index profile Δ n ( z (loc) , x ( ⊥ ) , t ) that it creates in the medium by, for example, Kerr effect, ionization, or plasma wave generation—evolve in complex, often unrepeatable, ways for which no single-shot recording method exists. Detailed knowledge of such evolving structures is essential for understanding, optimizing and scaling the myriad applications of laser- and particle-matter interactions, yet is available for individual shots only from computer simulations based on estimated initial conditions. Several methods to visualize laser- and particle-generated structures were developed previously. For example, ‘snapshot’ images of quasi-static ( t -independent) laser-generated structures Δ n ( z (loc) , x ( ⊥ ) ) (refs 11 , 12 )—analogous to Muybridge’s horse standing on a light-velocity treadmill—were produced using frequency-domain holography (FDH) [13] , [14] , in which a longitudinally stretched probe pulse (and a reference pulse with which it interfered in a spectrometer) copropagated with the object. Such images revealed relativistic curvature of quasi-linear plasma wake fronts [11] and resolved molecular and plasma contributions to formation of a stable laser filament in gas [12] . However, FDH snapshots blur if the objects evolve as they propagate. Thus, strongly nonlinear plasma wakes [15] yielded FDH snapshots [16] that averaged over time variations essential to their function [17] ; similarly, FDH cannot image the stochastic break-up of a pulse into multiple filaments. A frequency-domain streak camera (FDSC), in which the evolving object imprints a phase streak on an FDH-like probe pulse that crossed its path obliquely [18] , yielded partial single-shot information about the object’s evolution, but not a Muybridge-like image sequence. Motion-picture images of time-varying light-velocity objects have therefore been produced only by probing them transversely at different time delays over multiple shots [19] , [20] , [21] , analogous to strobing Muybridge’s horse over successive gallop cycles. One limit of this approach for light-velocity objects is that the transit time τ of a transverse probe pulse across the object’s width averages internal longitudinal structure of scale Δ z (loc) < vτ . Nevertheless, this approach has achieved impressive z (loc) resolution of very thin objects by using extremely short probe pulses. For example, Buck et al. [20] produced a shadowgraphic movie of plasma wakes of period Δ z (loc) <4 μm and width ~5 μm by probing transversely with ~6 fs pulses on successive shots. Nevertheless, the principal limit of multishot visualization is that it is not viable for non-repetitive or stochastic events typical of highly nonlinear interactions [2] , [15] , [21] , propagation in turbulent media [22] , or interactions driven by sources with low repetition rate [23] , unstable pointing, or other shot-to-shot fluctuations. Here we present a new approach to visualizing evolving light-velocity objects that yields a Muybridge-like movie sequence in one shot, enabling up to four-dimensional (4D) visualization of infrequent or stochastic laser- or particle-driven events for the first time, and greatly speeding visualization of events that are stable from shot to shot. The method utilizes multiple probe pulses, each an FDSC [18] crossing the object’s path at a different angle. However, the heart of the method is based on two key innovations that go well beyond FDSC. First, to avoid runaway complexity and cost, we developed compact, inexpensive methods to generate and detect multiple synchronized probe pulses. Instead of an unwieldy hyper-Michelson interferometer [24] , we generated the multiprobe array in a single step by cascaded four-wave mixing. On the detection side, instead of multiple expensive spectrometers, we multiplexed all probes to one spectrometer and extracted all phase streaks in one step from one high-information-density spectral hologram. Consequently, our apparatus is as simple and robust as a standard pump–probe experiment. Second, to transform phase streaks into a movie, we adapted established methods of computerized tomography [25] , [26] for the first time to reconstruct ultrafast spatiotemporal dynamics. We generalized the Radon transformation—conventionally used to reconstruct the spatial structure of a stationary object (for example, an internal bodily organ, underground petroleum reserve, or hidden manufacturing defect) from its projections, measured sequentially [25] or simultaneously [27] —to reconstruct both the spatial structure and the ultrafast temporal dynamics of an evolving light-velocity object. Similar to any optical visualization system, frequency-domain tomography (FDT) has resolution limits in z (loc) , x ( ⊥ ) and t . Instead of transit time, z (loc) resolution is limited by probe bandwidth, which can be increased as needed by supercontinuum generation [14] . As for a simple camera, x ( ⊥ ) resolution is limited by diffraction and lens aberrations. Finally, evolution time t resolution is limited to changes occurring over propagation distances z larger than the object’s dimensions, analogous to the paraxial approximation embedded in most mathematical treatments of nonlinear pulse propagation, yet allowing visualization of most dynamics of interest. 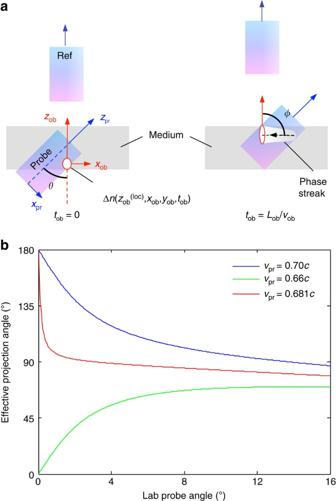Figure 1: Phase streak and projection angle. (a) Schematic of chirped probe pulse crossing path of evolving index object Δnat laboratory angleθ, producing phase streak at projection angleφ. Attob=0, the index object (red circle) overlaps with the right side of the probe profile and the probe keeps going untiltob=Lob/vobwhen it overlaps with the left side of the probe, leaving a phase streak across the probe. (b) Plot ofφversusθfor three different probe velocities, as indicated in legend. The object propagates atvob=0.68cin all three cases. Phase streaks and projection angles Figure 1a schematically depicts a single probe pulse of centre wavelength λ pr crossing the path of an evolving pump-generated object Δ n ( , x ob , y ob , t ob ) at laboratory angle θ , thereby accumulating phase streak ψ (θ) ( , x pr , y pr ) via cross-phase modulation. Here Δ n and ψ (θ) are expressed in the coordinates of the respective co-moving frames of object (ob) and probe (pr) pulses. We shall assume that the effective propagation length L eff over which any region of the probe profile overlaps the object is shorter than a probe diffraction length = π (Δ +Δ )/ λ pr n ( λ pr ), which is valid for the experiments presented below, and for a wide range of other interactions of interest (for example, laser-plasma accelerators in gas jets). Here, Δ x ob , Δ y ob are the object’s transverse radii, and L eff is less than the medium length L because the object drifts across the probe as they propagate at different angles and/or velocities. Diffraction of the probe pulse from the object can then be neglected, and its phase shift can be expressed as an integral Figure 1: Phase streak and projection angle. ( a ) Schematic of chirped probe pulse crossing path of evolving index object Δ n at laboratory angle θ , producing phase streak at projection angle φ . At t ob =0, the index object (red circle) overlaps with the right side of the probe profile and the probe keeps going until t ob = L ob / v ob when it overlaps with the left side of the probe, leaving a phase streak across the probe. ( b ) Plot of φ versus θ for three different probe velocities, as indicated in legend. The object propagates at v ob =0.68 c in all three cases. Full size image over the index object. In this limit, a point of the probe pulse accumulates a phase shift only when a linear chord of the object sweeps through it. Equation (1) is a 4D generalization of the Radon transform widely used in conventional tomography [25] . If diffraction is important, then equation (1) should be replaced with a Fresnel diffraction integral. To use equation (1), Δ n ( , x ob , y ob , t ob ) must be transformed from the coordinates of its own co-moving frame to those of the probe frame (see Methods). The Radon transform equation (1) then becomes: The phase streak (equation (2)) represents a projection of the index object in 4D space ( , x ob , y ob , t ob ) onto the three-dimensional (3D) probe profile space ( , x pr , y pr ). In conventional tomography, the projection angle is simply the laboratory angle θ at which probe light intersects the stationary object. In FDT, the projection angle φ ( θ ) differs from, but depends on, θ . φ is the angle between the object’s propagation direction and the axis of the phase streak (see Fig. 1a ). A straightforward derivation (see Methods) yields where the argument in brackets is a complex number of the form x + iy corresponding to angle φ =tan −1 ( y / x ) with the real axis. Figure 1b plots θ versus φ at different v pr for fixed v ob . As typically v ob ~ v pr for light-velocity index objects, a relatively narrow range of θ , which is convenient for laboratory set-up, can yield a broad range of φ , which optimizes image reconstruction quality. For example, for v ob =0.68 c and v pr =0.66 c , typical of an 800-nm pump and 400-nm probe in glass, equation (3) yields projection angle range −70°< φ <70° for probe angle range −10°< θ <10°. Projection angles φ =0 and π /2 have special meaning. A phase streak with φ =0 is obtained with θ =0 (co-propagating object and probe) and v ob > v pr (equivalently, φ = π corresponds to θ =0, v ob < v pr ). Such streaks reveal evolution of the object’s transverse ( x ( ⊥ ) ) profile, as it drifts longitudinally along the probe profile. Unlike FDH where velocity walk-off between co-propagating object and probe is a disadvantage because it blurs the image, in FDT it becomes an advantage because it creates a phase streak at φ =0 that is equivalent to streaks created by angular walk-off, and adds to the information pool for tomographic reconstruction. Streaks at φ ~ π /2 reveal evolution of the object’s longitudinal ( z (loc) ) profile as it drifts sideways across the probe profile. Optimal FDT reconstruction should include projection angles near both of these values. FDT movie reconstruction Each probe pulse carries a 3D projection (equation (2)) of the complete 4D object that is, in principle, fully recoverable. Below, however, we present recording procedures that select a two-dimensional (2D) slice of the phase streak in equation (2) at a desired constant y pr = y 0 . Thus, from here on, we outline the reduced procedure for recovering a tomographic movie of the 3D slice Δ n ( , x ob , y 0 , t ob ) from the selected 2D projections ψ (θ) ( , x pr , y 0 ) rather than the full 4D visualization. 4D imaging can be achieved by splitting the probes and sending copies to different spectrometers, each slicing a different y 0 . Of various conventional tomographic algorithms [25] , here we adapt algebraic reconstruction techniques (ARTs) [25] , [28] , [29] , because they are compatible with a smaller number of probes, are less susceptible to reconstruction artefacts and more readily incorporate independent knowledge of the object than other Radon-transform-based algorithms. ART is an iterative algorithm in which one guesses the object’s shape at each step, compares with measured projections, then modifies the guess until residuals are minimized (see Methods). In each iteration, independent information—for example, measured laser pulse profiles entering and exiting the medium and known optical properties of the medium—were incorporated and constrained trial solutions for Δ n . No prior assumptions about the object’s symmetry are made, in contrast to, for example, Abel inversions that assume cylindrical symmetry. FDT resolution limits The ability of FDT to resolve an evolving object Δ n ( , x ob , y 0 , t ob ) must be considered separately for each variable , x ob and t ob . Resolution of ‘intraframe’ ( , x ob ) structure at a given time t ob is determined by imaging optics and light-wave properties, as for conventional imaging of non-evolving objects. Wide probe bandwidth optimizes resolution. For example, to resolve non-evolving ~2 μm structures by FDH, supercontinuum probes were used [14] . Diffraction and lens aberrations determine x ob resolution of each frame. Single-element imaging lenses achieve ~5 μm resolution routinely. Aberration-corrected optics enable higher x ob resolution. The new criterion that enters with tomographic movies is ‘interframe’ time ( t ob ) resolution. FDT is designed to fully resolve objects that satisfy the paraxial approximation, that is, the drive pulse and its index object evolve slowly over propagation distances z ob of the order of the object’s dimensions. Thus, for an object of tens of microns longitudinal and lateral extent (typical of those created by a loosely focused ~100 fs laser pulse), picosecond-scale evolution is fully resolved. More rapid evolution is still observable, with limited resolution. Interframe resolution depends on the length of the phase streak relative to the object’s dimensions. FDT can resolve ~ N stages of the object’s temporal evolution, where N is the number of separated objects of dimensions ( , Δ x ob ) that can be lined up along the streak axis. Technical details and estimates of interframe resolution for experiments discussed below are presented in Methods. FDT image quality and reconstruction artefacts Image quality depends on the number and distribution of probes, and is quantified via the normalized root mean squared (RMS) deviation d (or ‘error’) of a reconstruction Δ n ( z (loc) , x , t ) from the evolving object Δ n 0 ( z (loc) , x , t ). We define d by generalizing its conventional 2D expression [25] , [26] to 3D: The z (loc) , x sums run over intraframe pixels, the t sums over frames and Δ is the object’s average index. The actual object Δ n 0 ( z (loc) , x , t ) is, of course, not directly accessible in a real tomographic reconstruction. Direct comparison of the reconstructed object with physical simulations and independent measurements are thus important for validating FDT reconstructions. In addition, d can be determined for a given probe configuration by simulating the reconstruction of a ‘phantom’ object that is known exactly. 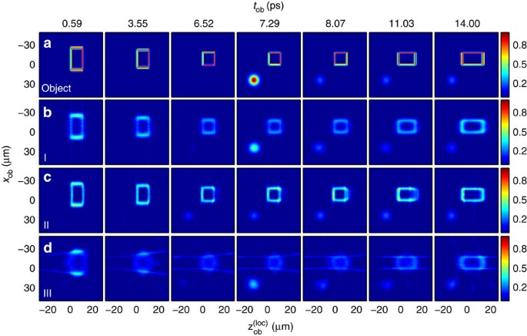Figure 2: Phantom simulations. (a) 2D snapshots (xobversus) of evolving ‘phantom’ object at seven selected timestobafter entering a medium (that is, seven locationszob=vobtobalong its propagation path) as it propagates with velocityvob=0.68c. The longitudinal axis of each snapshot indicates local distancefrom the centre of the object, with the object’s leading edge to the right. Remaining rows show tomographic reconstructions of the phantom object for three probe configurations: (b) Nineteen probes at projection angles −90°<φ<90° with 10° separation,vpr=0.70c(configuration I); (c) 18 probes at −90°<φ<80° with 10° separation,vpr=0.681c(configuration II); (d) 5 probes at −70°<φ<70° with 35° separation,vpr=0.66c(configuration III). The colour bar shows the dimensionless refractive index change of original and reconstructed objects. Phantom simulations Figure 2a shows selected 2D ( x ob versus ) snapshots of an artificial phantom index object at seven different times t ob (listed along the top) after entering a medium. These times correspond to object centre positions ranging from entrance ( z ob =0) to exit ( z ob =3 mm) of the medium. The horizontal spatial scale of each snapshot denotes , with the object’s leading edge (analogous to the head of Muybridge’s horse) to the right along the propagation direction z ob . The phantom does not evolve by a real physical process, although some of its general features (for example, propagation length, x ob and dimensions, evolution speed) were chosen to resemble those that occur in experiments below. The phantom’s detailed features were chosen to illustrate resolution limits, and to evaluate reconstruction artefacts, more effectively than a real physical process. Specifically, the object starts as a hollow rectangle with thin boundaries of widths Δ =2 μm (left and right) and Δ x 0 =5 μm (top and bottom), as shown by dotted curves in Fig. 3b,c , respectively. Such a thin rectangle separately and stringently tests transverse and longitudinal resolution limits. As it propagates at v ob =0.68 c , chosen to equal pump group velocity in experiments, the rectangle narrows along x ob over 0< t ob <7.3 ps, thus mimicking self-focusing observed in those experiments. During a short transition period ( t ob ~7.3±0.2 ps), a ‘dot’ of Gaussian profile appears to the lower left of the rectangle, quickly grows to Δ n max and falls to 0.2Δ n max ( Fig. 3a , dotted curve), mimicking the time scale of plasma generation and partial recombination in the experiments. As the dot grows within an interval (~100 fs) comparable to the object’s duration Δ / v ob , it tests interframe resolution. By breaking axial symmetry, it also tests the algorithm’s ability to reconstruct objects without prior assumptions about symmetry. The narrowed rectangle then expands longitudinally over 7.3 ps< t ob <14 ps, mimicking group-velocity stretching of a laser pulse. Figure 2: Phantom simulations. ( a ) 2D snapshots ( x ob versus ) of evolving ‘phantom’ object at seven selected times t ob after entering a medium (that is, seven locations z ob = v ob t ob along its propagation path) as it propagates with velocity v ob =0.68 c . The longitudinal axis of each snapshot indicates local distance from the centre of the object, with the object’s leading edge to the right. Remaining rows show tomographic reconstructions of the phantom object for three probe configurations: ( b ) Nineteen probes at projection angles −90°< φ <90° with 10° separation, v pr =0.70 c (configuration I); ( c ) 18 probes at −90°< φ <80° with 10° separation, v pr =0.681 c (configuration II); ( d ) 5 probes at −70°< φ <70° with 35° separation, v pr =0.66 c (configuration III). The colour bar shows the dimensionless refractive index change of original and reconstructed objects. 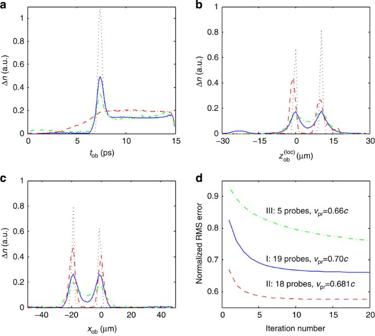Figure 3: Analysis of phantom simulations. (a) Peak Δnof the Gaussian ‘dot’ versus evolution timetob=zob/vob, demonstrating interframe resolution; (b,c) lineouts attob=7.3 ps (that is,zob=1.5 mm) of the rectangle along(b) andxob(c), demonstrating intraframe resolution. Curves ina–crefer to phantom simulations inFig. 2: original object (black dotted curve) and reconstructions with 19 (blue solid curve), 18 (red dashed curve) and 5 (green dash-dot curve) probes. (d) Normalized root mean square error of the same three tomographic reconstructions versus iteration number. Full size image Figure 3: Analysis of phantom simulations. ( a ) Peak Δ n of the Gaussian ‘dot’ versus evolution time t ob = z ob / v ob , demonstrating interframe resolution; ( b , c ) lineouts at t ob =7.3 ps (that is, z ob =1.5 mm) of the rectangle along ( b ) and x ob ( c ), demonstrating intraframe resolution. Curves in a – c refer to phantom simulations in Fig. 2 : original object (black dotted curve) and reconstructions with 19 (blue solid curve), 18 (red dashed curve) and 5 (green dash-dot curve) probes. ( d ) Normalized root mean square error of the same three tomographic reconstructions versus iteration number. Full size image Figure 2b–d shows tomographic reconstructions of the phantom from three probe configurations I through III. Figure 3a–c compares selected lineouts of the reconstructed images, with those of the object (dotted curves), whereas Fig. 3d plots RMS errors versus iteration number. In all cases, the probe bandwidth and imaging optics fully resolved the object’s intraframe ( z (loc) , x ) features. Variations among reconstructions I–III thus arose solely from different probe number, angular distribution and velocity as follows: (I) 19 probes each with v pr =0.70 c distributed equally over projection angles −90°< φ <90°; (II) 18 probes each with v pr =0.681 c distributed equally over −90°< φ <80°; (III) 5 probes each with v pr =0.66 c distributed equally over −70°< φ <70°. As expected, configurations I, II with 18–19 probes yielded sharper frame images of the slowly evolving rectangle ( Fig. 2b,c ) and sharper lineouts of its edges (blue and red curves, respectively, in Fig. 3b,c ), than the 5-probe configuration III, which yielded more blurred images with reconstruction artefacts ( Fig. 2d ) and less distinct edge lineouts (dashed green curves, Fig. 3b,c ). Reconstructions I and II also converged more rapidly towards smaller steady-state RMS error than configuration III ( Fig. 3d ). Thus, large probe number is one factor that promotes high-fidelity reconstruction of slowly evolving objects. On the other hand, all three configurations resolved the rectangle’s slow narrowing and lengthening equally well (see Fig. 2b–d ). Reconstructions of the ‘dot’ reveal more subtle comparisons. Configuration I, having the widest φ range and largest | v pr − v ob |=0.02 c , best resolved the dot’s ultrafast evolution ( Fig. 3a , blue curve), consistent with the discussion of FDT resolution above and in Methods. Configuration III, having the same | v pr − v ob | and similar φ range, resolved this feature nearly as well ( Fig. 3a , dashed green curve), despite only five probes. Configuration II, in contrast, failed completely to resolve it ( Fig. 3a , red curve), a consequence of its small | v pr − v ob |=0.001 c . Nevertheless, configuration II yielded sharper images of the rectangle ( Fig. 2c ) and smaller RMS error ( Fig. 3d ) than configuration I, despite one less probe. Evidently reduced blurring of slowly evolving objects is a compensating advantage of small | v pr − v ob |. Thus, in choosing | v pr − v ob |, an FDT system designer must compromise between resolving interframe evolution and minimizing intraframe RMS error. Experimental FDT setup and procedure As a laboratory demonstration of FDT, we visualized a 3D slice Δ n ( , x ob , y 0 , t ob ) of the evolving nonlinear refractive index envelope of a pump pulse (duration τ pu =100 fs, wavelength λ pu =800 nm, energy 0.4≤ E pu ≤0.7 μJ) focused with f -number ~30 to radius w 0 =25 μm (peak incident intensity 0.4≤ I 0 ≤0.7 TW cm −2 ) near the entrance of a Kerr medium: a fused silica plate of linear index n 0 ( λ pu )=1.45 and lowest-order Kerr coefficient n 2 ≈2 × 10 −16 cm 2 W −1 . Incident power exceeded the critical power P cr =3.7 /8 πn 0 n 2 ≈3.2 MW for self-focusing by a factor of 1.2 to 2.2. Our plate thickness L =3 mm satisfied the weak diffraction criterion L eff < L diff (pr) underlying equation (1). At our highest E pu , we observe a 3D slice of dynamics preceding self-guided filament formation [30] , [31] . The primary technical challenge in implementing FDT in the laboratory is to avoid runaway complexity and cost in generating, formatting and detecting a multiprobe pulse array. Conventional multiprobe experiments require an array of beam splitters to divide probes from pump, and a multimirror hyper-Michelson interferometer to format the probe train. Such setups are challenging to align and sensitive to vibrations. Moreover, recording the phase streaks by conventional FDH methods requires a separate spectrometer with charge-coupled device (CCD) detector for each probe. We addressed this challenge with the setup in Fig. 4 . Only two ‘probe-generating’ pulses (800 nm, 30 fs, 30 μJ) were split directly from the pump. These crossed simultaneously at a small adjustable angle ( α ~5 mrad) in a three-layer structure consisting of a β-barium borate (BBO) crystal sandwiched between two HZF4 glass plates. Cascaded four-wave mixing in the first HZF4 plate (5 mm thick, ~10 −15 cm 2 W −1 ) created a fan of up to eight 800 nm daughter pulses. The number depended on probe generator intensity and was limited by the onset of self-focusing and self-phase modulation. The BBO crystal (Type I, 500 μm thick) then frequency-doubled each beam and created an additional probe midway between each fundamental pair by sum-frequency generation, producing a fan of up to fifteen 400 nm probes separated from each other by angle α /2. The second HZF4 plate (15 mm thick) chirped them to 600 fs duration. Any desired subset of the array was easily selected by blocking unwanted probes. Here, for reasons discussed in Methods, we selected five probes at θ =0.1°, 1.4°, −1.2°, −7.6° and 9.5° inside the fused silica, corresponding to projection angles φ =1.0°, 27°, −25°, −65° and 68°, respectively, for v ob =0.68 c and v pr =0.66 c . 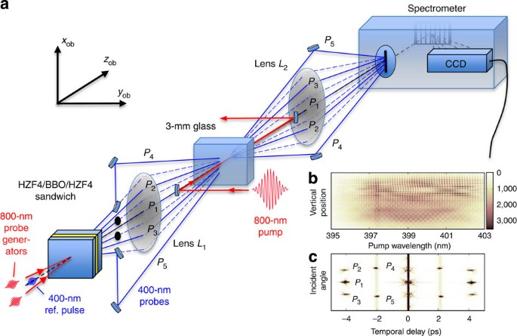Figure 4: Schematic set-up for single-shot FDT of evolving laser-generated structures. An 800-nm pump pulse of intensityI, coupled into and out of a glass slab by dichroic mirrors, creates an evolving luminal-velocity refractive index structure due to the nonlinear refractive indexn2Iand pump-generated plasma. Two probe-generating pulses split from the pump generate an array of chirped, frequency-doubled probe pulses in an HZF4/BBO/HZF4 sandwich. LensL1directs each probe across the pump path through the glass, where each acquires a phase streak that records evolution of the refractive index structure from a different angle. Optionally, selected probes can be diverted to angles beyond the optical aperture ofL1(see probesP4,P5), or blocked as shown (see dashed optical paths). LensL2images undeflected, unblocked probesP1–P3from the glass exit face to the entrance slit of an imaging spectrometer, which selects a slice of the projected image. Large-angle probesP4,P5were relayed by confocal lenses equivalent toL1and L2(not shown). The probes interfere inside the spectrometer with a temporally advanced 400 nm reference pulse, creating a 2D frequency domain hologram on a CCD at the spectrometer’s detection plane, shown inbfor five probes. Fourier transformation of this data yields a reciprocal hologram,c, in which peaksP1throughP5encode the phase modulations of the five probes. Phase streaks inFig. 5are recovered by windowing and inverse Fourier transforming these five peaks. Figure 4: Schematic set-up for single-shot FDT of evolving laser-generated structures. An 800-nm pump pulse of intensity I , coupled into and out of a glass slab by dichroic mirrors, creates an evolving luminal-velocity refractive index structure due to the nonlinear refractive index n 2 I and pump-generated plasma. Two probe-generating pulses split from the pump generate an array of chirped, frequency-doubled probe pulses in an HZF4/BBO/HZF4 sandwich. Lens L 1 directs each probe across the pump path through the glass, where each acquires a phase streak that records evolution of the refractive index structure from a different angle. Optionally, selected probes can be diverted to angles beyond the optical aperture of L 1 (see probes P 4 , P 5 ), or blocked as shown (see dashed optical paths). Lens L 2 images undeflected, unblocked probes P 1 – P 3 from the glass exit face to the entrance slit of an imaging spectrometer, which selects a slice of the projected image. Large-angle probes P 4 , P 5 were relayed by confocal lenses equivalent to L 1 and L 2 (not shown). The probes interfere inside the spectrometer with a temporally advanced 400 nm reference pulse, creating a 2D frequency domain hologram on a CCD at the spectrometer’s detection plane, shown in b for five probes. Fourier transformation of this data yields a reciprocal hologram, c , in which peaks P 1 through P 5 encode the phase modulations of the five probes. Phase streaks in Fig. 5 are recovered by windowing and inverse Fourier transforming these five peaks. Full size image Spatiotemporal overlap of multiple probes was achieved automatically by imaging the first HZF4 glass plate to the sample with lens L 1 ( f =20, 3 cm diameter). The pump-generated object swept across and imprinted a phase streak on each probe. To probe at angles θ beyond the aperture of L 1 , mirrors can re-direct selected probes from the fan along independent delivery lines to the sample. This was done for our two largest angle probes P 4 , P 5 . As shown in Fig. 4 , a chirped 400-nm reference pulse also split from the pump, co-propagated with it, advanced temporally by T ~2–4 ps. Lens L 2 ( f =15 cm, f -number 5.6) imaged reference and phase-modulated probes from the sample exit face to the slit of a single-imaging spectrometer, which selected a lineout of constant y 0 , thus limiting the final reconstructed objects to 3D slices Δ n ( , x ob , y 0 , t ob ) of the full 4D object Δ n ( , x ob , y ob , t ob ). Lens L 2 also ensured simultaneous, spatially overlapped delivery of all probes within its aperture. Reference and probes interfered inside the spectrometer, projecting a grid-like frequency-domain intensity pattern or hologram I ( ω , x ) ( Fig. 4b ) onto the CCD. This hologram stored the phase modulations of all probes in one shot, analogous to coherent multiplexing methods in holographic data storage [32] . To analyse phase shift in each probe, a 2D Fourier transform of I ( ω , x ) yielded a reciprocal 2D hologram Ĩ ( T , ) ( Fig. 4c ), in which each reference-probe interference pattern appeared as an isolated peak ( P 1 through P 5 ) at a position determined by probe angle and time-delay T . Peaks P 4,5 appear at a different T than other peaks because P 4 and P 5 have their own references (not shown). Each phase streak was reconstructed by windowing and inverse Fourier-transforming a specific peak P i , as in FDH. The peak P i must be well separated to avoid cross-talk. This requirement, together with the angular acceptance of the CCD and imaging optics, governed our selection of five probes (see Methods). Although this five-probe system adequately resolved the main self-focusing dynamics, a substantial increase in probe number and image quality is available by investing in large aperture, aberration-corrected lenses and a larger, more finely pixelated CCD. 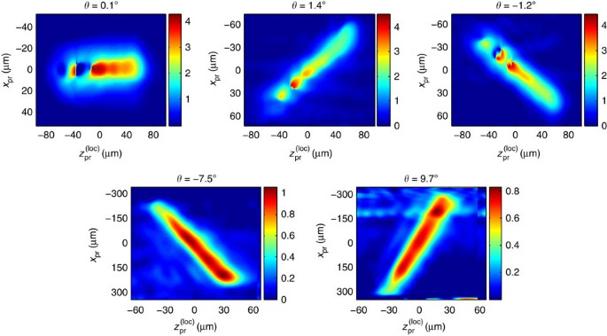Figure 5: Phase streaks induced by the evolving index profile. Epu=0.7 μJ and projection angles areφ=1.0°, 27°, −25° (top row), and −65° and 68° (bottom). Vertical (horizontal) scales denote transverse (longitudinal) position of the pump-induced phase streak within the temporally stretched probe pulse profile. The right-most end of each streak corresponds to the entrance of the medium;xpr==0 is approximately the midpoint of the pump pulse propagation through the Kerr medium. The spectrometer slit was centred on the images thatL2projected at the spectrometer entrance. Colour bars give phase shift in rad. Figure 5 shows five phase streaks for E pu =0.7 μJ. Small φ streaks (top row) highlight evolution of the object’s transverse ( x ob ) profile. Oscillations in transverse radius Δ x ob and peak index change Δ n max , indicating dynamic balance between self-focusing and defocusing, were evident in the last ~1/3 of these streaks. Streaks near φ ~70° (bottom row) highlight evolution of its longitudinal ( ) profile, which remained nearly constant due to the low dispersion of fused silica. To visualize evolution of the object’s full Δ n ( , x ob , y 0 , t ob ) profile, we tomographically reconstructed a movie from all five streaks using the ART algorithm [25] , [28] , [29] . Figure 5: Phase streaks induced by the evolving index profile. E pu =0.7 μJ and projection angles are φ =1.0°, 27°, −25° (top row), and −65° and 68° (bottom). Vertical (horizontal) scales denote transverse (longitudinal) position of the pump-induced phase streak within the temporally stretched probe pulse profile. The right-most end of each streak corresponds to the entrance of the medium; x pr = =0 is approximately the midpoint of the pump pulse propagation through the Kerr medium. The spectrometer slit was centred on the images that L 2 projected at the spectrometer entrance. Colour bars give phase shift in rad. 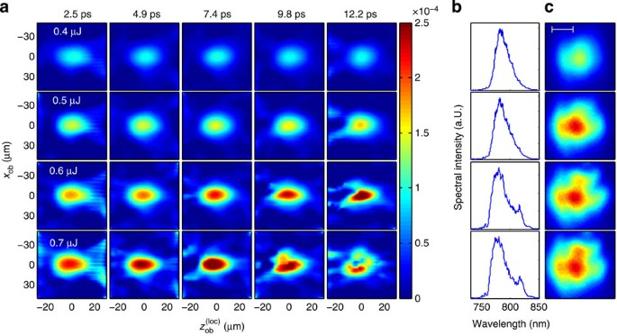Figure 6: Single-shot tomographic movies of the evolving index profile. (a) Selected 2D snapshots Δn(,xob) of the pump nonlinear index profile at five different propagation timestobindicated at the top and pump energies indicated at left. The horizontal axis of each snapshot is given in local position. The colour bar shows the dimensionless refractive index change. (b) Spectra of the transmitted pump pulses. The spectrum in the top row is nearly identical to the incident spectrum. (c) Near-field images of the transmitted pump spatial profiles, with a resolution of ~20 μm. Scale bar, 30 μm. Full size image Experimental movies of nonlinear laser propagation in glass Figure 6a shows movie frames, or 2D snapshots, of the nonlinear index profile Δ n ( , x ob ) at five selected propagation times t ob after entering ( t ob =0) and before exiting ( t ob =15 ps) the Kerr medium, for E pu from 0.4 μJ (top row) to 0.7 μJ (bottom row). The interframe spacing (Δ t ob =2.4 ps, Δ z ob =500 μm) approximates the interframe resolution limit for transverse profile variations and twice this limit for longitudinal variations. Supplementary Movie 1 shows continuously streaming movies with higher frame density. The main feature in each frame is a positive Δ n ( , x ob ) profile of transverse 1/ e 2 radius 13<Δ x ob <25 μm and longitudinal duration ~20 μm, or ~100 fs, that is attributable mainly to the instantaneous lowest-order nonlinear Kerr response n 2 I pu of fused silica to the pump pulse. Diffraction, characterized by length = π (Δ x ob ) 2 / λ pu n 0 ( λ pu ), and self-focusing, characterized by focal length L nl = λ pu /2 πn 0 n 2 I pu (ref. 33 ), respectively, govern most transverse pump dynamics. The reconstruction resolves them as long as >500 μm (that is, Δ x ob >14 μm) and L nl >500 μm (that is, I pu <1 TW cm −2 ). Self-focusing beyond these limits can introduce dynamics faster than the interframe resolution, as well as additional nonlinearities such as plasma generation [12] , [34] , [35] and higher-order Kerr effect [36] , [37] , [38] . Dispersion, characterized by length L dis = / β 2 =277 mm, governs evolution of the longitudinal profile [33] . As L dis ≫ L , the pulse and its n 2 I pu profile propagate with negligible change in duration. Figure 6: Single-shot tomographic movies of the evolving index profile. ( a ) Selected 2D snapshots Δ n ( , x ob ) of the pump nonlinear index profile at five different propagation times t ob indicated at the top and pump energies indicated at left. The horizontal axis of each snapshot is given in local position . The colour bar shows the dimensionless refractive index change. ( b ) Spectra of the transmitted pump pulses. The spectrum in the top row is nearly identical to the incident spectrum. ( c ) Near-field images of the transmitted pump spatial profiles, with a resolution of ~20 μm. Scale bar, 30 μm. Full size image The reconstructed movies in Fig. 6a depict various propagation regimes. For E pu =0.4 μJ (top row), Δ x ob and index shift Δ n ( =0, x ob =0) at the centre of the profile remained nearly constant over 15 ps (3 mm propagation distance), indicating that diffraction and self-focusing were balanced. For E pu =0.5 μJ (second row), Δ x ob contracted slightly, whereas Δ n (0, 0) increased slightly ( I pu increased from 0.5 to 0.6 TW cm −2 ), indicating that self-focusing slightly dominated. In these cases, the exit pump spectrum ( Fig. 6b , top two rows) and spatial profile ( Fig. 6c , top two rows) retained nearly their incident shapes (not shown), and transverse dynamics were fully resolved. At E pu =0.6 μJ, the pulse self-focused strongly and monotonically to Δ x ob ≈15 μm and I pu >1.5 TW cm −2 , indicating that self-focusing dynamics slightly exceeded the interframe resolution limit near the end of the medium. New structure developed in the output spectrum ( Fig. 6b , third row), a consequence of self-phase modulation, and in the spatial profile, which split into three lobes ( Fig. 6c , third row). The last movie frame shows the uppermost of these lobes separating from the central profile at t ob =12.2 ps ( z ob =2.5 mm), thus capturing the onset of multifilamentation. The other lobe lies outside the image plane. At E pu =0.7 μJ, similar structure developed in the exit spectrum and beam profile ( Fig. 6b,c , fourth row). In this case, however, the pulse self-focused to Δ x ob ≈15 μm ( I pu >1.5 TW cm −2 ) within 7.4 ps ( z ob =1.5 mm; Fig. 6a , fourth row) instead of 15 ps ( z ob =3 mm), after which further collapse was arrested and substructure developed in the index profiles. One such substructure is the split-off of the upper spatial lobe, now evident at t ob =9.8 ps ( z ob =2.0 mm). The dominant new feature, appearing at t ob =12.2 ps ( z ob =2.5 mm), is a steep-walled index ‘hole’ near the centre of the Δ n profile. No such ‘hole’ was observed in the exit beam profile ( Fig. 6c , fourth row). Thus, it is the result of a negative index change that locally cancels the positive nonlinear index change n 2 I pu . This feature appears within a single frame and thus, similar to the ‘dot’ in the phantom simulations of Fig. 2 , tests the interframe resolution of the tomographic reconstruction. To help understand the results in Fig. 6 , we calculated propagation of the pump using a nonlinear Schrödinger equation (NLSE) [30] , [31] that included diffraction, group-velocity dispersion, self-steepening, electronic and Raman-induced Kerr self-focusing, multi-photon and tunnelling ionization [39] , electron-hole recombination and plasma defocusing (see Methods). Input pulses were modelled as Gaussians that retained cylindrically symmetry as they propagated [30] , [31] . The calculations thus do not capture asymmetric multifilamentation observed in some FDT images, but adequately model propagation up to the formation of such filaments. 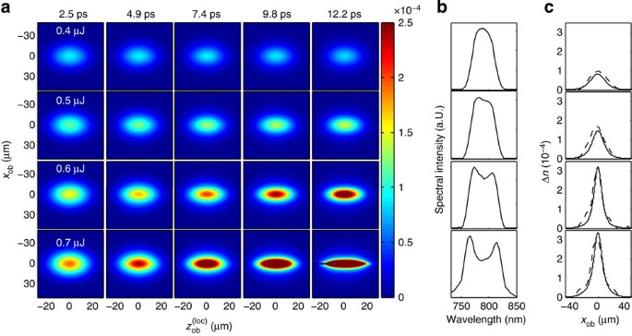Figure 7: NLSE-simulated movies of the evolving index profile. (a) Selected 2D snapshots Δn(,xob) of the pump nonlinear index profile from NLSE simulations for the same four pump energies and same five propagation times as shown inFig. 6a. The colour bar indicates the dimensionless refractive index change. (b) Spectra of the transmitted pump pulses from NLSE simulations, for direct comparison with measured spectra shown inFig. 6b. (c) Solid curves: NLSE-simulated pump transverse spatial profiles at=0 near the exit plane (tob=12.2 ps,zob=2.5 mm) for pump energy from 0.4 to 0.6 μJ, and attob=7.4 ps (zob=1.5 mm) for 0.7 μJ. Dashed curves: corresponding lineouts of FDT-reconstructed pump spatial profile fromFig. 6afor direct comparison. Figure 7a shows multiframe movies of the evolving Δ n ( , x ob , t ob ) from NLSE simulations neglecting high-order Kerr effect, for direct comparison with FDT reconstructions in Fig. 6a . Simulated and reconstructed movies agree with high fidelity despite the lack of any adjustable parameters. To quantify this agreement, Table 1 lists RMS deviations d between the FDT reconstructions in Fig. 6a and the NLSE simulations in Fig. 7a . For most frames of Fig. 6a , d ≤0.5, even smaller than for the 18–19 probe configurations of the phantom simulation (see Fig. 3d ). This reflects the high fidelity of these reconstructions, as well as the absence of sharp-edged structures that were inserted into the phantom simulations to test stringently for reconstruction artefacts. We observe d >0.5 in two places. First, frames that encompass the entrance ( t ob <2.5 ps, z ob <0.5 cm) or exit ( t ob >12.2 ps, z ob >2.5 mm) of the medium (not shown in Fig. 6a ) yield larger d because of ‘edge artefacts’ attributable to the sharp index discontinuity. When edge frames are omitted, we observe d <0.5 for 0.4≤ E pu ≤0.6 μJ (compare first and second rows of Table 1 ). Second, in the last two frames for E pu =0.7 μJ, we observe d >0.5. This is in part because the ‘real’ pulse develops multiple filaments ( Fig. 6c , bottom) that cylindrically symmetric NLSE simulations fail to capture, even though FDT reconstructions capture a slice of them. Thus, here a shortcoming of the NLSE simulation, not the FDT reconstruction, contributes to larger d . The small index ‘hole’ that appears at t ob =12.2 ps ( z ob =2.5 mm) also contributes, because it challenges FDT resolution in all three variables ( , x ob , t ob ) and deviates in shape from the narrower (in x ob ), longer (in ) negative-index plasma filament that appears in the corresponding NLSE simulation frame. Excluding these final two frames, d <0.5 even for E pu =0.7 μJ (third row of Table 1 ); including them, d exceeds that of the phantom five-probe configuration III (see Fig. 3d ) by only ~25%. Despite locally enhanced d , the reconstruction captures the essential physical feature (a transient plasma filament), albeit with distorted shape. Thus, direct comparison of Figs 6a and 7a and RMS error analysis show that the reconstructions are not significantly corrupted by artefacts. Figure 7: NLSE-simulated movies of the evolving index profile. ( a ) Selected 2D snapshots Δ n ( , x ob ) of the pump nonlinear index profile from NLSE simulations for the same four pump energies and same five propagation times as shown in Fig. 6a . The colour bar indicates the dimensionless refractive index change. ( b ) Spectra of the transmitted pump pulses from NLSE simulations, for direct comparison with measured spectra shown in Fig. 6b . ( c ) Solid curves: NLSE-simulated pump transverse spatial profiles at =0 near the exit plane ( t ob =12.2 ps, z ob =2.5 mm) for pump energy from 0.4 to 0.6 μJ, and at t ob =7.4 ps ( z ob =1.5 mm) for 0.7 μJ. Dashed curves: corresponding lineouts of FDT-reconstructed pump spatial profile from Fig. 6a for direct comparison. Full size image Table 1 RMS deviations of FDT reconstructions from NLSE simulations. Full size table Figures 7b,c , 8 and 9 highlight several specific areas of quantitative agreement. First, regarding transverse profiles, Fig. 8 compares (a) Δ x ob ( t ob ) (full width at half maximum) and (b) Δ n (0,0, t ob ) from reconstructions (data points) with NLSE-simulated values (solid curves). For E pu =0.4, 0.5 μJ, they agree well for all t ob ; for E pu =0.6, 0.7 μJ, they agree up to the onset of multifilamentation, beyond which solid calculated curves are drawn dotted. Figure 7c directly compares the complete simulated (solid curves) and reconstructed (dashed) transverse index profiles near the exit plane (for E pu =0.4, 0.5, 0.6 μJ) or at the onset of multifilamentation (0.7 μJ), further illustrating the close agreement. Second, both simulated ( Fig. 7a ) and reconstructed ( Fig. 6a ) longitudinal profiles evolve negligibly ( Fig. 9a ) and agree with independent autocorrelation measurements ( Fig. 9b ) of incident and transmitted pulse duration, as expected for L << L dis . Although longitudinal breakup of the pulse temporal envelope (‘pulse splitting’) triggered by material dispersion [33] , [40] or ionization [30] , [41] has been observed in previous fs pulse filamentation experiments and simulations, and is an important mechanism in arresting self-focusing collapse [5] , our NLSE simulations predict that pulse splitting would occur only for z ob >0.3 cm (for E pu =0.7 μJ), beyond our sample length. Previous observations of fs pulse splitting in glass used higher power pulses [30] or longer propagation lengths [33] than our experiment. Third, simulated ( Fig. 7b ) and measured ( Fig. 6b ) output pump spectra show similar trends as E pu increases. Specifically, the simulations reproduce the development of an asymmetric double-peaked spectrum for E pu ≥0.6 μJ, caused by self-phase modulation. The asymmetry in the peaks is attributable to slight self-steepening, which otherwise plays a minor role, as our sample length L is much less than the characteristic self-steepening length L ss = cτ pu / n 2 I pu ≈15 cm (ref. 42 ) for our conditions. 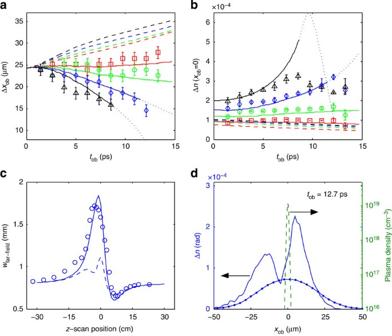Figure 8: Comparison of FDT data with NLSE simulations. (a) Reconstructed radius Δxoband (b) index shift Δn(=0,xob=0) at the centre of Kerr profiles Δn(=0,xob=0) fromFig. 6aversus propagation timetob. Data points are for variousEpu: red squares, 0.4 μJ; green circles, 0.5 μJ; blue diamonds, 0.6 μJ; black triangles, 0.7 μJ. ForEpu=0.7 μJ andtob>8.8 ps, Δxobis not well defined because of the complex Kerr profile shape, and thus is not plotted. Solid curves are from NLSE calculations taking onlyn2Ipuinto account; the dotted portion of these curves indicates the region after multiple filaments formed. Dashed curves include fourth-order Kerr effect withn4=−3.3 × 10−28cm4W−2(ref.36). Error bars inaare equal to the vertical axis pixel size of each movie frame inFig. 6aand denote error in measuringxob. Error bars inbare the maximum difference of index shift within interframe temporal resolution Δtob. (c) Results ofz-scan measurements of Kerr lensing by the fused silica plate. Data points show far-field beam radius downstream of the silica plate placed at indicated timetobfrom the vacuum waist of 100 fs pulses focused tow0=120 μm,I0=0.6 TW cm−2in vacuum. Solid blue curve is calculated radius based on lowest-order Kerr lensing, dashed curve includesn4as above. (d) Lineout (solid blue curve) of Δnversusxobat=0,tob=12.7 ps (zob=2.6 mm), showing index hole near centre of the Kerr profile, compared with calculated radial distribution of plasma density (dashed curve) attob=12.7 ps (zob=2.6 mm) due to six-photon ionization. Calculated peak plasma density overestimates actual peak density by as much as 26because calculatedIpuoverestimates actualIpuatzob=12.7 ps (zob=2.6 mm) by ~2 (compare black dotted curve and data points inb). Dotted blue curve shows suppression of the Kerr profile from fourth-order Kerr effect usingn4as above. Figure 8: Comparison of FDT data with NLSE simulations. ( a ) Reconstructed radius Δ x ob and ( b ) index shift Δ n ( =0, x ob =0) at the centre of Kerr profiles Δ n ( =0, x ob =0) from Fig. 6a versus propagation time t ob . Data points are for various E pu : red squares, 0.4 μJ; green circles, 0.5 μJ; blue diamonds, 0.6 μJ; black triangles, 0.7 μJ. For E pu =0.7 μJ and t ob >8.8 ps, Δ x ob is not well defined because of the complex Kerr profile shape, and thus is not plotted. Solid curves are from NLSE calculations taking only n 2 I pu into account; the dotted portion of these curves indicates the region after multiple filaments formed. Dashed curves include fourth-order Kerr effect with n 4 =−3.3 × 10 −28 cm 4 W −2 (ref. 36 ). Error bars in a are equal to the vertical axis pixel size of each movie frame in Fig. 6a and denote error in measuring x ob . Error bars in b are the maximum difference of index shift within interframe temporal resolution Δ t ob . ( c ) Results of z -scan measurements of Kerr lensing by the fused silica plate. Data points show far-field beam radius downstream of the silica plate placed at indicated time t ob from the vacuum waist of 100 fs pulses focused to w 0 =120 μm, I 0 =0.6 TW cm −2 in vacuum. Solid blue curve is calculated radius based on lowest-order Kerr lensing, dashed curve includes n 4 as above. ( d ) Lineout (solid blue curve) of Δ n versus x ob at =0, t ob =12.7 ps ( z ob =2.6 mm), showing index hole near centre of the Kerr profile, compared with calculated radial distribution of plasma density (dashed curve) at t ob =12.7 ps ( z ob =2.6 mm) due to six-photon ionization. Calculated peak plasma density overestimates actual peak density by as much as 2 6 because calculated I pu overestimates actual I pu at z ob =12.7 ps ( z ob =2.6 mm) by ~2 (compare black dotted curve and data points in b ). Dotted blue curve shows suppression of the Kerr profile from fourth-order Kerr effect using n 4 as above. 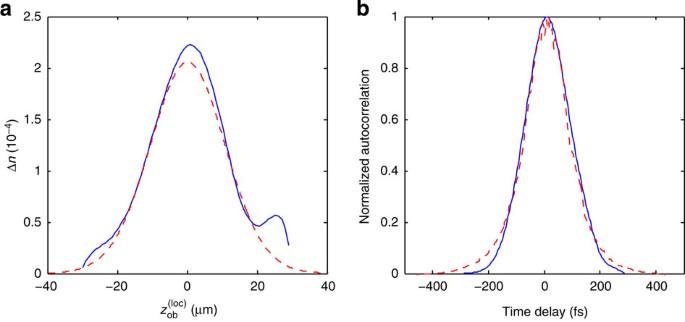Figure 9: Direct comparison of measured and calculated longitudinal pulse profiles. (a) FDT reconstruction (blue solid line) and NLSE simulation (red dashed line) of the longitudinal profile. (b) Autocorrelation trace calculated from FDT-reconstructed longitudinal profile (blue solid line) and direct measurement (red dash line). Except for the direct autocorrelation measurement, the curves are lined out fromFigs 6and7withtob=7.4 ps,xob=0 andEpu=0.6 μJ. Full size image Figure 9: Direct comparison of measured and calculated longitudinal pulse profiles. ( a ) FDT reconstruction (blue solid line) and NLSE simulation (red dashed line) of the longitudinal profile. ( b ) Autocorrelation trace calculated from FDT-reconstructed longitudinal profile (blue solid line) and direct measurement (red dash line). Except for the direct autocorrelation measurement, the curves are lined out from Figs 6 and 7 with t ob =7.4 ps, x ob =0 and E pu =0.6 μJ. Full size image Beyond the point at which 0.6, 0.7 μJ pumps lost cylindrical symmetry, the calculations, although no longer in quantitative agreement with the data, nevertheless mirror qualitative trends in the FDT images. For example, for E pu =0.7 μJ and t ob >9.8 ps ( z ob >2.0 mm), the calculated Δ n (0, 0, t ob ) increases sharply to ~0.00065 before dropping equally sharply ( Fig. 8b , black dotted curve) due to formation of an electron-hole plasma, which contributes a compensating negative index change. The measured Δ n (0, 0, t ob ) increases to a lower maximum, then also drops ( Fig. 8b , black data points). Here the calculated Δ n evolves more quickly than the interframe resolution; thus (like the ‘dot’ in the phantom simulations), the reconstruction ‘rounds off’ the temporal or z ob dynamics, partly explaining the discrepancy. Absence of multifilamention in the calculation also contributes to the discrepancy. The FDT images themselves provide additional insight. In this region, the steep-walled index ‘hole’ appeared (see Fig. 6a , bottom right frame), inducing de-focusing and presumably pulse splitting in a longer medium [30] , [33] , [40] , [41] . This hole had ~10 μm diameter, significantly narrower than the n 2 I pu envelope (see Fig. 8d , solid curve). Such a narrow hole is consistent with the onset of multiphoton ionization, the mechanism that accounts for the drop in Δ n (0, 0, t ob ) in our NLSE simulation. Six photons are needed to create an electron-hole pair in fused silica; hence, the plasma generation rate scales as I 6 . Thus, plasma concentrates in the centre of the self-focused profile ( Fig. 8d , dashed curve) and appears suddenly as I increases, consistent with the FDT images. Possible additional contributions to this feature are discussed in Methods. In summary, we have demonstrated a single-shot tomographic method for visualizing spatiotemporal dynamics of light-velocity objects. Compact methods to generate and detect multiple synchronized probe pulses were demonstrated, Radon transformation methods were adapted to recovery of motion pictures and image-quality limits were elucidated through phantom simulations and laboratory experiments. FDT can image a wide range of nonlinear propagation phenomena, including filament formation in gases and the evolution of plasma wakefields. Derivation of projection angle To express the generalized Radon transform in the form of equation (2), it is necessary to relate object to probe coordinates. To do so, we first define stationary lab frame coordinates ( t i , x i ′, y i ′, z i ′), where i = (ob, pr) and the z i ′ axis is parallel to the propagation direction of the object or probe pulse. For pulses propagating in the x – z plane, these coordinates are related by: z ob ′= z pr ′cos θ + x pr ′sin θ and x ob ′=− z pr ′sin θ + x pr ′cos θ . We then apply canonical transformations ( , x i , y i , t i )=( z i ′− v i t , x i ′, y i ′, t i ) between lab and pump/probe co-moving frames, where v i is the velocity of the object or probe pulse, to obtain and the inverse relations where we use t ob = t pr . Equation (5) immediately yield the arguments of the integrand in equation (2). To derive equation (3) relating φ to θ , define the starting point of the streak axis as the common origin of − x pr and − x ob coordinate systems at t ob =0. The former origin moves to ( , x ob ) in the latter system at t ob >0, thereby defining the streak axis. Once the phase-modulated probe propagates into free space, where it is detected, these coordinates become ( c / v ob , x ob ), yielding which becomes equation (3) on substituting equation (5) with =0 and x pr =0. Similarly, the starting and end points of the streak axis have coordinates (0, 0) and ( , x pr ), respectively, in − x pr coordinates. The components of the streak length vector are thus Δ = and Δ x pr = x pr , which yields equation (8) on substituting equation (6) with =0 and x ob =0 and putting L = v ob t ob . FDT interframe resolution limits The length of a phase streak at probe angle θ is , where are the two components of the streak length vector for an object propagating through a medium of length L . Thus, transverse profile evolution, measured using small θ probes, is best resolved when . As Δ ∝ | v pr − v ob | at small θ , using pump and probe pulses with a large velocity mismatch optimizes transverse temporal resolution. Longitudinal profile evolution, measured using large θ probes, is best resolved when . As Δ x pr ∝ sin θ , including probes up to θ max = θ ( φ ≈ π /2) optimizes longitudinal resolution. As a numerical example relevant to the experiments, for which v ob =0.68 c , v pr =0.66 c , Δ =20 μm, Δ x ob =50 μm and θ max = θ ( φ =70°)=14°, the temporal resolution is ~( v pr / v ob )Δ /| v ob − v pr |≈3 ps and ~Δ x ob /( v ob sin θ max )≈1 ps for transverse ( T ) and longitudinal ( L ) profile evolution, respectively. Interframe resolution is thus determined by probes at the extreme angles 0 and θ max , but does not depend on the number or angular distribution of probes between these angles. Angular distribution of probes The distribution of probe angles is a key FDT design feature, in addition to those discussed in the main text. For designs with equivalent probe number and | v pr − v ob |, an even angular distribution of probes with maximized φ range yields the smallest RMS error, analogous to the limit-angle problem of conventional computerized tomography [25] . Absence of | φ |>70° probes in configuration III (see ‘Phantom simulations’ section of main text), illustrates this point. The absence introduces streak artefacts into the reconstructed profiles ( Fig. 2d ). The artefacts persist, and RMS error remains above that of configurations I, II even when probe number within | φ |≤70° is the same as in those configurations (not shown). Experimental limits on the maximum probe number In general, the maximum number of probe N is limited by the peak separation in Fig. 4c , which is related to the angular separation Δ θ between probes. In the experiment, Δ θ was limited to the probe divergence angle Δ θ min = λ pr /Δ x ob , or ~10 mrad for our system. On the other hand, the spectrometer CCD pixel size x pix ~40 μm limited the maximum probe-reference angular separation to θ max = Mλ pr / x pix ~200 mrad, where M ~20 is the magnification of lens L 2 . Thus, ideally our system supports N max = θ max /Δ θ min ~20. In practice, θ max is limited to ~100 mrad (and N max to ~10) by the physical aperture and spherical aberration of lenses L 1 and L 2 . We chose Δ θ conservatively at ~2Δ θ min to thoroughly eliminate cross-talk, yielding five probes. ART movie reconstruction On the basis of equation (2), each pixel value ψ i of a 2D phase streak was obtained by applying a linear projection operator P on the 3D tomographic movie voxels Δ n j : Following ART, we applied an iterative procedure to solve equation (9) by setting initial solution Δ =0 and updating this solution to fit the measured phase streak ψ i in the k th iteration via where λ =0.1 is the relaxation parameter for ART iterations. When the 2D projections ψ (θ) ( , x pr , y 0 ) contained 2 π jumps, a 2D phase unwrapping pre-processing procedure was applied to the measured phase ψ i through the weighted minimum norm algorithm [43] . Simulations Pump pulse propagation was simulated using the model in ref. 31 , in which an NLSE and a coupled electron-hole plasma generation-recombination equation were solved numerically. where ζ= z (loc) / v . In the NLSE, the first and second terms are responsible for transverse diffraction and longitudinal dispersion, respectively, and the third nonlinear term N NL = ik 0 n 2 T [(1− f R )| A | 2 + f R R (ζ) ⊗ | A (ζ)| 2 ] A − (1+ iω 0 t c ) T −1 ( ρA )− A denotes instantaneous Kerr effect, delayed Raman-induced Kerr effect, plasma absorption/defocusing and photo-ionization loss of the laser wave. We also performed some simulations that included a fourth-order Kerr term n 4 term, as discussed in the next section. The operator T =1+( i / ω 0 )∂/∂ζ leads to self-steepening and space-time coupling. The plasma generation-recombination equation has taken photo-ionization, avalanche ionization and recombination into account, whereas the photo-ionization term W PI (| A | 2 ) is based on Keldysh’s formulation generalizing both multiphoton and tunnelling ionization mechanisms [39] . To compare simulation results with experimental data, transverse (longitudinal) imaging resolution Δ x res ~5 μm ( / v ob ~70 fs) were taken into account by convolving the simulated index profile with a Gaussian function with transverse (longitudinal) dimension Δ x res ( / v ob ). Simulation parameters were either from our direct measurements (for example, n 2 =2 × 10 −16 W cm −2 from z -scan measurements) or most recent references for each parameter: n 4 =−3.3 × 10 −28 W cm −2 (ref. 36 ); n 0 =1.45, group velocity dispersion β 2 =36.1 fs 2 mm −1 , silica band gap E g =9 eV and constants τ d =32 fs, τ s =12 fs, f R =0.18 for the Raman response function R (ζ) = τ s exp(−ζ/ τ d )sin(ζ/ τ s ) [31] ; plasma collision time τ c =1.7 fs and plasma recombination time τ r =170 fs (ref. 44 ). High-order Kerr effect The relative importance of plasma defocusing [12] , [34] , [35] and negative electronic Kerr effect [36] , [37] , [38] in arresting the collapse of self-focusing pulses has been debated extensively in connection with nonlinear pulse propagation in gaseous media. Although there has been comparatively little discussion of this issue for condensed media, a measured value n 4 =−3.3 × 10 −28 cm 4 W −2 of the fourth-order Kerr coefficient of fused silica has been reported [36] . In view of this measurement, and the importance of nonlinear pulse propagation in fused silica in optical fibre communication and micro-machining, we considered the possibility that fourth-order Kerr effect might contribute to, or even dominate, the arrest of self-focusing under our conditions. There were three findings. First, our NLSE calculations that included fourth-order Kerr effect using the previously reported n 4 deviated significantly from all FDT data, even before the onset of multifilamentation, as shown by the dashed curves in Fig. 8a,b of the main text. This n 4 actually induced self-defocusing under our conditions, contrary to observation. RMS deviation d between the NLSE calculations and the reconstructions ( Fig. 6a ) also grew to >0.8, even in regions free of edge artefacts and for E pu ≤0.6 μJ, much larger than values in Table 1 . Second, as an independent check of | n 4 / n 2 |, we conducted standard z -scan measurements of our silica plate’s nonlinear index [45] . Results, exemplified by Fig. 8c of the main text (circles), fit well to a nonlinear lens determined solely by n 2 I pu (solid curve). Our FDT and z -scan results both place an upper limit of 10 −29 cm 4 W −2 on | n 4 |. Third, we found that a negative 4th-order Kerr effect, even of limited value, broadly suppressed the positive n 2 I pu profile, rather than producing the observed narrow index hole that appeared at t ob =12.2 ps ( z ob =2.5 mm) for E pu =0.7 μJ (see Fig. 6a , fourth row, last panel). This is because it scales as instead of , as plasma generation does. Thus, our results do not support an important role of a fourth-order Kerr effect. However, they do not rule out the possibility that a negative electronic Kerr effect of higher than fourth order contributes to forming this index hole. How to cite this article: Li, Z. et al. Single-shot tomographic movies of evolving light-velocity objects. Nat. Commun. 5:3085 doi: 10.1038/ncomms 4085 (2014).